Designed synthesis of large-pore crystalline polyimide covalent organic frameworks Covalent organic frameworks (COFs) are an emerging class of porous crystalline polymers with a wide variety of applications. They are currently synthesized through only a few chemical reactions, limiting the access and exploitation of new structures and properties. Here we report that the imidization reaction can be used to prepare a series of polyimide (PI) COFs with pore size as large as 42 × 53 Å 2 , which is among the largest reported to date, and surface area as high as 2,346 m 2 g −1 , which exceeds that of all amorphous porous PIs and is among the highest reported for two-dimensional COFs. These PI COFs are thermally stable up to 530 °C. We also assemble a large dye molecule into a COF that shows sensitive temperature-dependent luminescent properties. Covalent organic frameworks (COFs) [1] , [2] , [3] , [4] are porous crystalline polymers and show promise for applications in gas storage [5] , [6] , semiconductive and photoconductive devices [7] , [8] , energy storage [9] and heterogeneous catalysis [10] , [11] . The key to COFs’ crystallinity is reversible bond formation during polymerization, without which amorphous porous polymeric materials form [12] , [13] , [14] . Owing to the challenging nature of reversible synthesis, COF materials can be achieved only with a limited number of organic reactions, namely boronic acid trimerization [15] , [16] , boronate ester formation [17] , [18] , Schiff base reaction [19] , [20] and nitrile trimerization [21] , [22] . Recently, Wuest and co-workers demonstrated another reaction, the nitroso self-addition [23] , by which diamondoid azodioxy networks could be obtained. To broaden the application and structural diversity of COF materials, introduction of new reactions is highly desired. The imidization reaction is typically used to produce polyimide (PI) polymers, which are known for high thermal stability, good chemical resistance and outstanding mechanical properties and are used widely in the electronics and semiconductor industry [24] . Recently, amorphous but intrinsically microporous aromatic PIs were synthesized, featuring spirobifluorene units as a structure directing motif [25] , [26] , [27] . These porous PIs exhibit the good thermal stability typical of PIs, but their surface area is limited, and in particular, non-uniform pore size limits their applications. Crystalline porous PIs have yet to be reported. In this study, we design and synthesize a series of large-pore crystalline PI COFs (termed PI-COFs) by achieving reversible imidization. These crystalline porous materials feature large pores whose size can be tuned by extending the building units. The 42 × 53 Å 2 channel size of PI-COF-3 is among the largest reported to date [28] and its 2,346 m 2 g −1 Brunauer-Emmett-Teller (BET) surface area exceeds that of all amorphous porous PIs and is among the highest reported for two-dimensional (2D) COFs. These PI-COFs show excellent thermal stability. In addition, PI-COF-3 is loaded with large dye molecules. The product shows distinctive temperature-dependent luminescent properties, suggesting that dye-doped COF materials can be used in temperature-sensing devices. Design of PI-COFs Our strategy for preparing new large-pore COFs involves imidizing the extended aromatic dianhydride and triamine building units. In the model condensation reaction of phthalic anhydride with aniline, one water is eliminated to yield an imide product, N -phenylphthalimide ( Fig. 1a ) [29] . On the basis of this reaction, the phthalic anhydride is extended to a linear building unit, pyromellitic dianhydride (PMDA), whereas aniline is extended to triangular building units of various sizes, such as tris(4-aminophenyl)amine (TAPA, 7 Å), 1,3,5-tris(4-aminophenyl)benzene (TAPB, 9 Å) or 1,3,5-tris[4-amino(1,1-biphenyl-4-yl)]benzene (TABPB, 13 Å), as measured from the molecular centre to the amine nitrogen ( Supplementary Fig. 1 ). As shown in Fig. 1b , the condensation reaction of PMDA and TAPA will give a 2D crystalline COF with 33 Å hexagonal pores, termed PI-COF-1. Replacing TAPA with larger amines produces different 2D crystalline COFs with larger hexagonal pores: for TAPB, the product is PI-COF-2 (37 Å, Fig. 1c ), and for TABPB, the product is PI-COF-3 (53 Å, Fig. 1d ). By linking the linear and triangular building units through the imidization reaction, the products are most likely 2D structures based on the boron nitride net (bnn, Fig. 1e ) [30] . 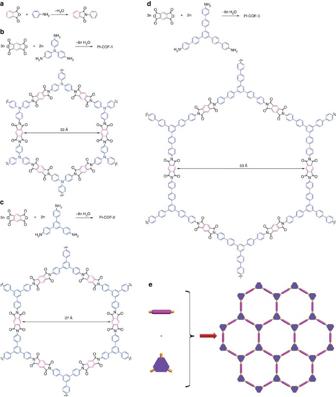Figure 1: Strategy for preparing large-pore crystalline polyimide COFs. (a) The model reaction between phthalic anhydride and aniline forms an imide monomer,N-phenylphthalimide. (b) Condensation of the extended dianhydride, pyromellitic dianhydride (PMDA) and the extended triamine tris(4-aminophenyl)amine (TAPA) gives a 2D crystalline polyimide COF with pore size of 33 Å, termed PI-COF-1. (c) Condensation of PMDA and the extended triamine 1,3,5-tris(4-aminophenyl)benzene (TAPB) forms a 2D crystalline polyimide COF with pore size of 37 Å, termed PI-COF-2. (d) Condensation of PMDA and the extended triamine 1,3,5-tris[4-amino(1,1-biphenyl-4-yl)]benzene (TABPB) produces a 2D crystalline polyimide COF with pore size of 53 Å, termed PI-COF-3. (e) Condensation of linear and triangular building units gives a 2D structure based on the boron nitride net (bnn). Figure 1: Strategy for preparing large-pore crystalline polyimide COFs. ( a ) The model reaction between phthalic anhydride and aniline forms an imide monomer, N -phenylphthalimide. ( b ) Condensation of the extended dianhydride, pyromellitic dianhydride (PMDA) and the extended triamine tris(4-aminophenyl)amine (TAPA) gives a 2D crystalline polyimide COF with pore size of 33 Å, termed PI-COF-1. ( c ) Condensation of PMDA and the extended triamine 1,3,5-tris(4-aminophenyl)benzene (TAPB) forms a 2D crystalline polyimide COF with pore size of 37 Å, termed PI-COF-2. ( d ) Condensation of PMDA and the extended triamine 1,3,5-tris[4-amino(1,1-biphenyl-4-yl)]benzene (TABPB) produces a 2D crystalline polyimide COF with pore size of 53 Å, termed PI-COF-3. ( e ) Condensation of linear and triangular building units gives a 2D structure based on the boron nitride net (bnn). Full size image Synthesis and characterization Typically, PI-COFs were synthesized by suspending PMDA with TAPA, TAPB or TABPB in a mixed solution of N -methyl-2-pyrrolidone (NMP), mesitylene and isoquinoline followed by heating at 200 or 250 °C for 5–7 days, giving crystalline solid at yields of 80% for PI-COF-1, 82% for PI-COF-2 and 63% for PI-COF-3 based on PMDA ( Supplementary Figs 2–4 ). These products were insoluble in water and common organic solvents, such as acetone, ethanol, hexanes, tetrahydrofuran (THF), N , N -dimethylformamide and m -cresol. To make the imidization reaction reversible, it is important to adjust the ratio of the solvents, use a suitable isoquinoline as catalyst and carry out the polymerization at an appropriate temperature. These conditions are fundamentally different from those used in the previous synthesis of amorphous porous PIs, where the monomers were completely solubilized, and thus quickly and irreversibly polymerized into amorphous materials [31] . The mixed solvent used here controls the solubility of the monomers, the suitable catalyst adjusts the speed of reactions, and the appropriate temperature promotes the imide ring-closing reactions. Fourier transform infrared ( Supplementary Figs 5–7 ) spectra showed absorptions at 1,774 and 1,720 cm −1 for PI-COF-1, 1,778 and 1,722 cm −1 for PI-COF-2 and 1,779 and 1,718 cm −1 for PI-COF-3, corresponding to asymmetric and symmetric vibrations, respectively, of C=O groups of the five-membered imide rings; whereas peaks at 1,375 cm −1 for PI-COF-1, 1,371 cm −1 for PI-COF-2 and 1,382 cm −1 for PI-COF-3 are attributed to the stretching vibration of the C–N–C moiety. Furthermore, no bands appeared corresponding to the starting monomers (amino around 3,340 cm −1 and anhydride at 1,765 cm −1 ) or amic acid intermediate (amide around 1,650 cm −1 ), demonstrating that the products are fully imidized networks. Solid-state 13 C cross-polarization magic-angle-spinning nuclear magnetic resonance (NMR) spectra ( Supplementary Fig. 8 ) confirmed the carbonyl carbon of imide ring at 163.6 p.p.m. for PI-COF-1, 165.3 p.p.m. for PI-COF-2 and 164.9 p.p.m. for PI-COF-3. The overlapping peaks from 114.3 to 144.6 p.p.m. are assigned to phenyl carbons. Under the present polymerization conditions, carbonyl signal for the amic acid group around 176 p.p.m. does not appear, suggesting that once the amino and anhydride react to yield the amic acid intermediate, the subsequent imide ring-closing reactions are completed immediately. Similar to amorphous porous PIs, these PI-COFs also showed high thermal stability as determined by thermogravimetric analysis (TGA): up to 520 °C for PI-COF-1, 535 °C for PI-COF-2 and 530 °C for PI-COF-3 ( Supplementary Figs 9–11 ). Crystalline structural resolution The crystallinity and unit cell parameters of the PI-COFs were determined by powder X-ray diffraction (PXRD) analysis ( Fig. 2 ). Considering complementary electron-rich and electron-poor π surfaces and the significant low-pressure nitrogen adsorption uptake in 2D COFs [32] , extended structures based on a serrated stacking bnn net in the space group of C mcm (no. 63), in which adjacent sheets were slipped by ¼ of the unit cell distances, were modelled for PI-COFs with the Materials Studio software package [33] . After a geometrical energy minimization using the universal force field, the unit cell parameters were obtained ( a =32.95 Å, b =57.07 Å, c =6.24 Å for PI-COF-1; a =37.24 Å, b =64.50 Å, c =6.25 Å for PI-COF-2 and a =52.59 Å, b =90.91 Å, c =6.15 Å for PI-COF-3). Simulated PXRD patterns were obtained in excellent agreement with the experimental ones ( Fig. 2 ). Furthermore, the full profile pattern matching (Pawley) refinements were carried out from the experimental PXRD patterns. Peaks at 3.10°, 5.36°, 6.20°, 8.20° and 10.8° for PI-COF-1; 2.75°, 4.75°, 5.50°, 7.25° and 9.50° for PI-COF-2 and 1.95°, 3.35°, 3.90°, 5.15° and 6.75° for PI-COF-3 correspond to the (110), (200), (220), (310) and (400) Bragg peaks of an orthorhombic lattice, respectively. The refinement results yield unit cell parameters nearly equivalent to the predictions with good agreement factors ( a =32.86 Å, b =57.01 Å, c =6.29 Å, wR p =7.53%, R p =4.21% for PI-COF-1; a =37.32 Å, b =64.52 Å, c =6.23 Å, wR p =7.77%, R p =4.56% for PI-COF-2 and a =52.62 Å, b =90.99 Å, c =6.15 Å, wR p =7.92%, R p =4.81% for PI-COF-3). We also considered alternative structures wherein adjacent sheets are eclipsed based on the space group of P 6/mmm (no. 191) or staggered based on the space group of P 6 3 /mmc (no. 194). For the eclipsed structures, the simulated PXRD patterns also agreed with the experimental patterns; however, the high gas uptake observed at low-pressure is less consistent with such structures. For the staggered structures, the simulated PXRD patterns did not match the experimental data ( Supplementary Figs 12–23 and Supplementary Tables 1–9 ). 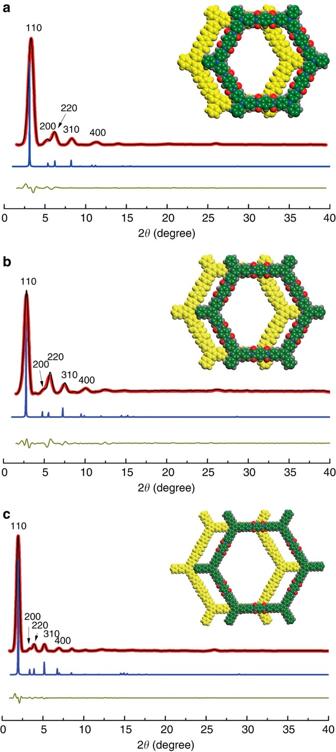Figure 2: Powder X-ray diffraction patterns of PI-COFs. (a–c) PXRD patterns of PI-COFs 1 to 3 with observed in black, refined in red, calculated based on the serrated stacking bnn net in blue, and the difference (observed minus refined profiles) in dark yellow. Inset: serrated stacking layers of PI-COFs 1 to 3, respectively. Figure 2: Powder X-ray diffraction patterns of PI-COFs. ( a – c ) PXRD patterns of PI-COFs 1 to 3 with observed in black, refined in red, calculated based on the serrated stacking bnn net in blue, and the difference (observed minus refined profiles) in dark yellow. Inset: serrated stacking layers of PI-COFs 1 to 3, respectively. Full size image On the basis of the above results, extended architectures of PI-COFs are proposed to be based on a serrated stacking bnn net with adjacent sheets slipped by ¼ of the unit cell distances ( Fig. 3a–d ). As the size of the triangular building unit increases from PI-COF-1 to PI-COF-3, the void volume becomes greater (35%, 41% and 55%), pore size larger (7 × 20 and 27 × 33 Å 2 , 9 × 24 and 29 × 37 Å 2 , and 11 × 30 and 42 × 53 Å 2 ; Supplementary Figs 24–26 ) and crystal density smaller (0.64, 0.55 and 0.39 g cm −3 ). The void volume and crystal density were calculated from crystal structure data. The pore size is defined as the distance between two opposite edges in the pore cross-section. The pore dimension in PI-COF-3 (42 × 53 Å 2 ) exceeds those of most open COF materials [34] and is among the largest reported for COFs, such as HHTP-DPB COF [35] with 47 Å and D TP -A PyrDI -COF [29] with 53 Å. 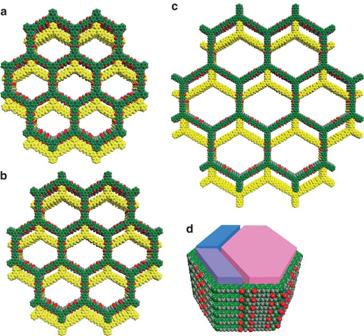Figure 3: Structural representations of PI-COFs. (a–c) Extended structure of PI-COFs 1 to 3, respectively. (d) Microporous (blue, purple) and mesoporous (pink) channels in PI-COF-3. C, green; H, grey; N, blue; O, red. Figure 3: Structural representations of PI-COFs. ( a – c ) Extended structure of PI-COFs 1 to 3, respectively. ( d ) Microporous (blue, purple) and mesoporous (pink) channels in PI-COF-3. C, green; H, grey; N, blue; O, red. Full size image Gas adsorption The architectural stability and porosity of PI-COFs were determined by measuring nitrogen gas (N 2 ) adsorption at 77 K, revealing reversible type-IV isotherms with a sharp uptake below P / P 0 =0.05 ( Fig. 4 ). The significant adsorption at low pressure supports the presence of micropores, whereas the step observed at P / P 0 =0.10–0.20 or 0.10–0.40 indicates pore condensation in mesopores with a narrow distribution. The absence of hysteresis during desorption is a common feature of materials containing hexagonally aligned 1D mesopores [36] . The presence of both micropores and mesopores is consistent with the serrated stacking bnn net with adjacent sheets slipped by ¼ of the unit cell distances. The total pore volumes were evaluated at P / P 0 =0.90 to be V p =0.53 cm 3 g −1 for PI-COF-1, 0.67 cm 3 g −1 for PI-COF-2 and 1.34 cm 3 g −1 for PI-COF-3. Pore size distributions of PI-COFs were calculated on the basis of nonlocal density functional theory. Large pores of width 29 Å for PI-COF-1, 33 Å for PI-COF-2 and 51 Å for PI-COF-3 dominate the distribution, and simultaneously small pores of about 21 Å for PI-COF-1, 20 Å for PI-COF-2 and 36 Å for PI-COF-3 can be observed, which is in agreement with pore sizes predicted from the crystal structures ( Fig. 4 , inset). The BET model was applied over the 0.05< P / P 0 <0.14 range of the isotherm, yielding BET surface areas of 1,027 m 2 g −1 for PI-COF-1, 1,297 m 2 g −1 for PI-COF-2 and 2,346 m 2 g −1 for PI-COF-3 ( Supplementary Figs 27–29 ). The surface area of PI-COF-3 is among the highest reported for 2D COFs, such as COF-10 5 with S BET =1,760 m 2 g −1 and ILCOF-1 (ref. 37 ) with S BET =2,723 m 2 g −1 , and exceeds those reported for amorphous porous PIs, such as MPI-1 (ref. 38 ) with S BET =1,454 m 2 g −1 and Td-PPI [39] with S BET =2,213 m 2 g −1 . 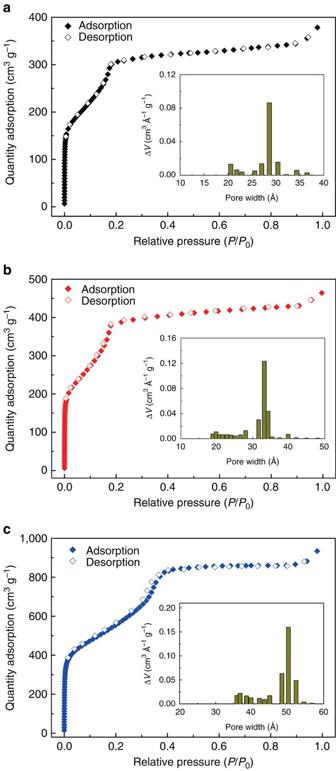Figure 4: Nitrogen gas adsorption and desorption isotherms for PI-COFs. (a) PI-COF-1; (b) PI-COF-2 and (c) PI-COF-3. Inset: pore size distribution of PI-COFs from fitting the nonlocal density functional theory (NLDFT) model to the adsorption data. Figure 4: Nitrogen gas adsorption and desorption isotherms for PI-COFs. ( a ) PI-COF-1; ( b ) PI-COF-2 and ( c ) PI-COF-3. Inset: pore size distribution of PI-COFs from fitting the nonlocal density functional theory (NLDFT) model to the adsorption data. Full size image Encouraged by the excellent stability and high porosity of this series of new COFs, we assembled a large organic molecule, rhodamine B (RB, 10 × 16 Å 2 , Supplementary Fig. 30 ), inside the COF with the largest channels, PI-COF-3. RB is a typical dye used extensively in biotechnology applications, exhibiting strong visible absorption and a high fluorescence quantum yield [40] , [41] . A number of studies have explored the incorporation of dye molecules into the channels of porous materials, such as mesostructured silica [42] and large-pore metal-organic frameworks [43] , owing to their potential applications in solid-state lasers, optical filtres and optoelectronics. However, such exploration has not been extended to COF materials. COFs constructed from strong covalent bonds between light elements have extra-large pores, excellent stability and lower refractive index, and thus dye-doped COFs are expected to be a more promising optical or sensor material. Typically, dye-doped PI-COF-3 was obtained by immersing PI-COF-3 in 1.0 × 10 −3 M RB in methanol for 24 h followed by filtration and washing. The resultant PXRD peaks coincide with those of the starting material, which confirms the structural integrity of dye-doped PI-COF-3 ( Supplementary Fig. 31 ). A nitrogen adsorption isotherm at 77 K of dye-doped PI-COF-3 indicated a slight decrease in N 2 adsorption because of the presence of RB molecules in the pores ( Supplementary Fig. 32 ). The dye-doping experiment was also repeated with RB solutions of higher concentrations (2.0 × 10 −3 and 4.0 × 10 −3 M). Fluorescence spectra of dye-doped PI-COF-3 were recorded at all three RB concentrations at room temperature ( Fig. 5a and Supplementary Figs 33 and 34 ). At 1.0 × 10 −3 M of RB, the strongest emission peak was at 594 nm with the excitation peak at 562 nm, which is similar to previous results for RB-doped hybrid materials [44] . At higher RB concentrations (2.0 × 10 −3 M and 4.0 × 10 −3 M), the emission peaks exhibited a red shift (from 594 to 601 and 609 nm, respectively, Fig. 5b ), indicating that the dye was present as fluorescent dimers (J-dimers) in the pores of PI-COF-3 (ref. 45 ). To confirm that the dye was present inside the pores, we prepared a sample in which dye molecules were intentionally only adsorbed on the surface by immersing PI-COF-3 in 1.0 × 10 −3 M RB in methanol for only 15 min followed by filtration without washing. Compared with the pore-loaded samples, which were prepared by stirring for 24 h followed by filtration and washing with anhydrous methanol, the surface-loaded sample showed a broader red-shifted fluorescence peak (from 594 to 603 nm, Supplementary Fig. 35 , curve b). More importantly, the surface-adsorbed dye molecules could be completely removed by washing with anhydrous methanol, after which no fluorescence was observed ( Supplementary Fig. 35 , curve c). Furthermore, the amount of RB in the pores of PI-COF-3 for different adsorption times was detected by TGA, showing a gradually increasing uptake of RB with increasing adsorption time ( Supplementary Figs 36 and 37 ). We also studied temperature dependence in the emission spectra ( Fig. 5c ). At 4.0 × 10 −3 M RB, the peak at 609 nm remained at the same location but increased linearly in intensity as temperature decreased from 298 to 77 K ( Fig. 5c , inset), a desirable property for applications in temperature-sensing devices. 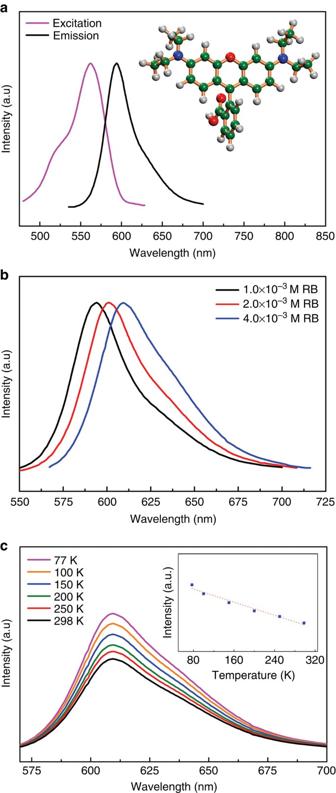Figure 5: Fluorescence spectra of dye-doped PI-COF-3. (a) Excitation and emission spectra at room temperature of PI-COF-3 doped in 1.0 × 10−3M RB solution in methanol for 24 h. Inset: molecular structure of RB. C, green; H, grey; N, blue; O, red. (b) Emission spectra at room temperature of PI-COF-3 doped in RB solutions with different RB concentrations for 24 h. (c) Emission spectra at different temperatures of PI-COF-3 doped in 4.0 × 10−3M RB solution in methanol for 24 h. Inset: change of fluorescence intensity with temperature. Figure 5: Fluorescence spectra of dye-doped PI-COF-3. ( a ) Excitation and emission spectra at room temperature of PI-COF-3 doped in 1.0 × 10 −3 M RB solution in methanol for 24 h. Inset: molecular structure of RB. C, green; H, grey; N, blue; O, red. ( b ) Emission spectra at room temperature of PI-COF-3 doped in RB solutions with different RB concentrations for 24 h. ( c ) Emission spectra at different temperatures of PI-COF-3 doped in 4.0 × 10 −3 M RB solution in methanol for 24 h. Inset: change of fluorescence intensity with temperature. Full size image In conclusion, we have synthesized a series of novel COFs by using the imidization reaction. The PI-COFs have large pore sizes that can be tuned by extending the building units, and in particular, PI-COF-3 displays a channel size among the largest reported to date. These PI-COFs show remarkable thermal stability and higher surface area than amorphous porous PIs. Furthermore, large dye molecules are loaded into COFs and the dye-doped PI-COF-3 exhibits clear temperature-dependent photoluminescence. The PI-COFs prepared in this work may not only expand COFs to an important class of polymers, PIs, but may also facilitate the development of dye-doped porous materials for applications in temperature-sensing devices. Synthesis of TABPB To a 100-ml three-neck round bottom flask was added 4-aminophenylboronic acid pinacol ester (1.10 g, 5.0 mmol), 1,3,5-tris(4-bromophenyl)benzene (0.80 g, 1.5 mmol), and Pd(PPh 3 ) 4 (10.0 mol%, 0.12 g) followed by 35.0 ml THF and 20.0 ml of 2 M K 2 CO 3 solution. The flask was degassed for 30 min before the solution was allowed to reflux under argon for 24 h. After addition of approximately 50.0 ml H 2 O, the product was extracted with CH 2 Cl 2 . The organic phase was eluted with THF and hexane through a silica column, then dried to yield a light yellow powder of TABPB (0.52 g, 60%; ref. 46 ). 1H NMR (400 MHz, DMSO- d 6 ) δ : 7.86, 7.82, 7.66, 7.43, 6.69, 5.72; 13 C NMR (400 MHz, DMSO- d 6 ) δ : 148.9, 141.9, 140.5, 137.9, 127.9, 127.7, 127.5, 126.3, 124.0, 114.9. Infrared (KBr): 3,448, 3,356, 3,205, 3,028, 1,616, 1,589, 1,497, 1,446, 1,389, 1,277, 1,180, 1,118, 810, 694, 571, 536, 505 cm −1 . Synthesis of PI-COF-1 A Pyrex tube measuring o.d. × i.d.=10 × 8 mm 2 was charged with PMDA (32.7 mg, 0.15 mmol) and TAPA (29.0 mg, 0.10 mmol) in a solution of 0.50 ml mesitylene/0.50 ml NMP/0.05 ml isoquinoline. The tube was flash frozen at 77 K (LN 2 bath), evacuated to an internal pressure of 0.15 mm Hg and flame sealed. Upon sealing the length of the tube was reduced to ca 13 cm. The reaction mixture was heated at 200 °C for 5 days to afford a brown precipitate, which was isolated by filtration over a medium glass frit and washed with anhydrous THF (20.0 ml). The product was immersed in anhydrous THF (20.0 ml) for 8 h, during which the activation solvent was decanted and replaced four times. The solvent was removed under vacuum at 80 °C to afford PI-COF-1 as a brown powder (45.1 mg, 80%). Anal. Calcd for C 66 H 30 N 8 O 12 : C, 70.34; H, 2.68; N, 9.94. Found: C, 70.22; H, 2.61; N, 10.02. Solid-state 13 C NMR (500 MHz) δ : 163.6, 144.6, 136.3, 127.9, 124.6, 114.3. Infrared (KBr): 1,774, 1,720, 1,603, 1,504, 1,375, 1,321, 1,269, 1,176, 1,119, 1,086, 922, 810, 721, 621, 526 cm −1 . Synthesis of PI-COF-2 In a manner similar to the preparation of PI-COF-1, treatment of PMDA (32.7 mg, 0.15 mmol) and TAPB (35.1 mg, 0.10 mmol) in a solution of 0.50 ml mesitylene/0.50 ml NMP/0.05 ml isoquinoline at 200 °C for 5 days afforded a brown precipitate (51.2 mg, 82%) after purification by the above-described method. Anal. Calcd for C 78 H 36 N 6 O 12 : C, 75.00; H, 2.90; N, 6.73. Found: C, 75.03; H, 2.81; N, 6.64. Solid-state 13 C NMR (500 MHz) δ : 165.3, 142.1, 136.4, 126.3, 117.8. Infrared (KBr): 1,778, 1,722, 1,597, 1,508, 1,444, 1,371, 1,176, 1,124, 1,014, 814, 721, 617, 561, 526 cm −1 . Synthesis of PI-COF-3 In a manner similar to the preparation of PI-COF-1, treatment of PMDA (32.7 mg, 0.15 mmol) and TABPB (58.0 mg, 0.10 mmol) in a solution of 0.50 ml mesitylene/0.05 ml NMP/0.05 ml isoquinoline at 250 °C for 7 days afforded a brown precipitate (54.2 mg, 63%) after purification by the above-described method. Anal. Calcd for C 114 H 60 N 6 O 12 : C, 80.27; H, 3.55; N, 4.93. Found: C, 80.20; H, 3.53; N, 4.91. Solid-state 13 C NMR (500 MHz) δ : 164.9, 141.7, 136.1, 125.2, 116.4. Infrared (KBr): 1,779, 1,718, 1,606, 1,553, 1,491, 1,382, 1,367, 1,286, 1,198, 1,113, 993, 912, 854, 800, 627, 523 cm −1 . Dye-doped PI-COF-3 Typically, PI-COF-3 was doped with large dye molecules by adding PI-COF-3 powder (0.50 g) to solutions of RB in 10 ml anhydrous methanol with different concentrations (1.0 × 10 −3 , 2.0 × 10 −3 or 4.0 × 10 −3 M). The mixtures were allowed to stir for 24 h to afford pink precipitate, which was isolated by filtration over a medium glass frit and washed with anhydrous methanol (20.0 ml). The solvents were removed under vacuum at 80 °C to produce dye-doped PI-COF-3. The results of PXRD and N 2 adsorption confirmed structural integrity of PI-COF-3 after dye assembly. The amounts of RB in PI-COF-3 after immersion in 1.0 × 10 −3 , 2.0 × 10 −3 or 4.0 × 10 −3 M for 24 h were determined by TGA to be 0.6 wt%, 0.9 wt% and 1.4 wt%, respectively ( Supplementary Fig. 38 ). The specifics of the calculation are as follows. The TGA results showed that the weight loss of pure RB began at 200 °C ( Supplementary Fig. 39 ). The amount of RB in PI-COF-3 could be determined by assuming the weight loss before 200 °C was from the residual methanol solvent and taking the loss from 200 to 300 °C as the weight loss from the decomposition of RB molecules, which is 17 wt% of the total RB weight as determined in Supplementary Fig. 39 . Although PI-COF-3 has a high free volume (16,153 Å 3 per unit cell) and is capable of loading more RB molecules (up to about 47 wt% based on a theoretical calculation), low incorporation is preferred because at high concentrations the dye forms non-fluorescent RB dimers (H-dimers), thus quenching excited states by a Foster type energy transfer [44] . Characterization 1 H NMR spectra were recorded on a Bruker AV 400 MHz spectrometer (Bruker). Solid-state 13 C NMR spectra were recorded on a Bruker AVIII 500 MHz spectrometer. Fourier transform infrared spectra were recorded on a Thermo Nicolet Nexus 470 spectrometer equipped with a MCT-A (mercury cadmium telluride) detector with 5 mg samples. TGA was carried out under nitrogen atmosphere on a TGA/DSC 1 thermal analyzer from METTLER TOLEDO. Elemental analyses were carried out on a Perkin-Elmer 240C element analyzer (Perkin-Elmer). PXRD data were collected on a Philips X’Pert powder diffractometer (Philips) using a Cu Kα source ( λ =1.5418 Å) over the range of 2 θ =1.0−40.0 with a step size of 0.02° and 2 s per step. Fluorescence spectroscopy data were collected on a LS55 luminescence spectrometer. The sorption isotherm for N 2 was measured with a Micromeritics ASAP 2020 analyzer with ultra-high-purity N 2 (99.999% purity). To estimate pore size distributions for PI-COFs, nonlocal density functional theory was applied to analyse the N 2 isotherms on the basis of the model of N 2 @77K on carbon with slit pores and the method of non-negative regularization. The scanning electron microscopy images were obtained on a JEOL JSM7400F microscope (JEOL), operating at an acceleration voltage of 3–10 keV and current of 10 μA. How to cite this article: Fang, Q. et al . Designed synthesis of large-pore crystalline polyimide covalent organic frameworks. Nat. Commun. 5:4503 doi: 10.1038/ncomms5503 (2014).